Graphenes in the absence of metals as carbocatalysts for selective acetylene hydrogenation and alkene hydrogenation Catalysis makes possible a chemical reaction by increasing the transformation rate. Hydrogenation of carbon–carbon multiple bonds is one of the most important examples of catalytic reactions. Currently, this type of reaction is carried out in petrochemistry at very large scale, using noble metals such as platinum and palladium or first row transition metals such as nickel. Catalysis is dominated by metals and in many cases by precious ones. Here we report that graphene (a single layer of one-atom-thick carbon atoms) can replace metals for hydrogenation of carbon–carbon multiple bonds. Besides alkene hydrogenation, we have shown that graphenes also exhibit high selectivity for the hydrogenation of acetylene in the presence of a large excess of ethylene. Catalysis is aimed at increasing the rate of chemical reactions. There are many reactions that would not occur in the absence of catalysts. Most of the catalysts use transition or heavy metals as active sites. Owing to the limited resources of some of these metals, it is of considerable importance to find alternatives that could be sustainable and more affordable than the present catalysts containing metals. Carbocatalysis, in which a material containing exclusively or predominantly carbon element in the absence of any metal is acting as a catalyst, is emerging as a promising area aimed at replacing traditional catalysts based on metals [1] , [2] , [3] , [4] . When the carbocatalysts are prepared from natural biopolymers, as the sample presented here, they are examples of environmental benignity and sustainability. In the context of carbocatalysis, the use of graphene (Gr) and related materials, such as graphene oxide (GO), are under the spotlight because of their large-scale availability and the various possibilities that these materials offer to introduce active sites [5] , [6] , [7] , [8] , [9] , [10] . Since the pioneer study by Bielawsky and co-workers [11] in 2010 showing that GO is an efficient catalyst for the aerobic oxidation of benzylic hydrocarbons, Gr-based materials are increasingly used as carbocatalysts for reactions such as aerobic oxidations and acid catalysis [12] , [13] , [14] , [15] , [16] , [17] , [18] . To validate the concept of carbocatalysis and demonstrate its generality and potential, the challenge is to prove that carbocatalysts based on Gr can compete as catalysts for reactions that are paradigmatically catalysed by transition metals. Hydrogenation of multiple C–C bonds is one of the most prominent examples of catalytic reactions carried out at large scale in petrochemistry and industry, but still requiring precious (Pt, Pd and Rh) or transition metals (Ni and Fe) as catalysts. Promoting hydrogenations with metal-free catalysts has turned out to be challenging; however, a significant progress in this area has been in the last 8 years with the development of rigid molecules with Lewis acid–base pairs at appropriate distance to activate molecular H 2 (refs 19 , 20 , 21 ). It would be important to show that carbocatalysts based on Gr materials in the absence of metals are also able to catalyse hydrogenation of multiple C–C bonds. There are scattered recent precedents reporting hydrogenation of ethylene and nitro aromatics with carbon materials. Although hydrogenation of Gr to form graphane is well documented [22] , [23] , [24] and has attracted interest as a preparation method of new Gr-based materials, up to now the possibility to use Gr as catalyst to activate molecular hydrogen has remained unexplored. One computational study has proposed based on calculations that zig-zag edges at the periphery of Gr having dangling bonds should strongly interact with molecular hydrogen, while armchair edges are not appropriate for hydrogen activation [25] . In addition, theoretical models predict that B-doped Gr should be able to interact with molecular hydrogen [26] . There is only one precedent on the hydrogenation of ethylene using reduced GO (rGO), but the reaction required very high temperatures (500 °C) and hydrogen excess to proceed, observing no conversion at 200 °C and only 3.2% at 250 °C, making the process uninteresting from the practical point of view [27] . With these precedents in mind, here we prepare a systematic series of Gr-based materials and test their ability to act as catalyst for hydrogenation reactions that can be taken as representative model compounds of important gas-phase and liquid-phase processes showing the generality of the process. The results obtained here are rationalized based on strong hydrogen adsorption on Gr sheets that is experimentally followed by thermoprogrammed hydrogen desorption measurements, H 2 /D 2 scrambling and on the existence of Lewis acid–base pairs able to interact with H 2 . Overall, the results presented here constitute an example of carbocatalysis showing the potential of this concept to replace very costly precious metals by low-value Gr materials. Gr preparation and characterization In the initial stage of our work, we proceeded to the preparation of the series of Gr materials that will be subsequently evaluated as carbocatalysts in hydrogenation reactions. 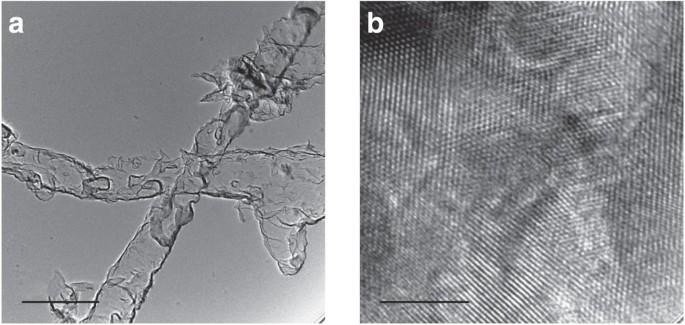Figure 1: Microscopy images. TEM (a, scale bar 500 nm) and HR-TEM (b, scale bar 5 nm) images recorded for (P)Gr showing the sample layer morphology from the contrast with the background, the characteristic wrinkles, the ordering and arrangement at the atomic level. Table 1 lists the materials prepared, the precursor, the preparation procedures and the heteroatom loading. The list includes GO that has been obtained starting from graphite by conventional Hummers oxidation to graphite oxide, followed by exfoliation by ultrasounds [28] . Considering the instability of GO in the presence of reducing agents including hydrogen, we also tested rGO obtained by thermal reduction of GO in water at 150 °C in an autoclave. The other Gr-based materials tested were obtained by pyrolysis of natural biopolymers modified or not by the presence of Na 2 HPO 4 . It should be noted that while GO is prepared using a large excess of permanganate and may contain some Mn residues in trace amounts (see below), the Gr materials obtained by pyrolysis have not been purposely in contact with any transition metal that could be responsible for the catalysis. Table 1 Hydrogenation catalysts with indication of precursor and preparation method. Full size table The preparation of these Gr-based materials has been already reported, and firm characterization data can be found in the literature [29] , [30] , [31] . Briefly, preparation of Gr consists of pyrolysis under inert atmosphere at 900 °C of commercial alginate that has been previously purified by dissolving it in water, filtering insoluble residues and recovering the purified solubilized alginate by evaporation. Nitrogen-doped Gr ((N)Gr) was obtained similarly by pyrolysis at 900 °C under inert atmosphere of commercial chitosan that was also purified from other residues by dissolution in aqueous acetic acid and filtration. P-doped Gr ((P)Gr) was obtained by adding a given amount of Na 2 HPO 4 to purified alginate in solution before obtaining an intimate mixture of Na 2 HPO 4 and alginic acids that was submitted to pyrolysis at 900 °C. Sulfur-doped Gr was obtained by pyrolysis at 1,000 °C of λ-carragenan that simultaneously acts as Gr precursor and as the source of S element. Powders of GO and rGO can be easily suspended in water and organic solvents using ultrasonication to form single or few-layer platelets of micrometric size as it is well known in the literature [32] . In addition, we have reported that turbostratic carbon residues resulting from pyrolysis of unmodified and modified alginate and chitosan afford, upon ultrasonication of water, methanol, dichlorometane and other organic solvents, few-layer two-dimensional (2D) graphenic platelets of dimensions about 2 μm or smaller [31] . The presence of the dopant elements was quantified by elemental combustion chemical analysis of C, N and S and by calibrated X-ray photoemission spectroscopy (XPS) analysis. All the samples exhibit almost coincident Raman spectra consisting of the 2D, G and D peaks appearing approximately at 2,500, 1,580 and 1,350 cm −1 , respectively. The relative intensity of the D peak compared with the G band gives a quantitative indication of the presence of defects and doping on the Gr-based materials. The observation of the D band in the Raman spectra of Gr obtained by pyrolysis of alginate and in rGO is because of the presence of some residual oxygenated functional groups, while for the rest of the samples is also because of the presence of dopant elements. The fact that all the doped Gr samples exhibit similar value for the relative intensity of the D band versus that of G indicates that the doped Gr samples should have similar vibrational properties and density of defects. Deconvolution of the XPS C1 s peak shows in general a predominant component at 284.5 eV attributable to sp 2 carbons of Gr, accompanied by other components in lesser proportions assigned to carbon atoms bonded to the dopant element and to oxygen. The dopant elements are responsible for the presence of the corresponding XPS peaks in a calibrated intensity that is in accordance with the proportion of this element and that can be deconvoluted in three, two and two components in the case of nitrogen (pyridinic, pirrolic and N-oxide), phosphorous (phosphine and phosphine oxide contributions) and sulfur (graphitic C–S–C and sulfoxide C–S–O), respectively. Supplementary Fig. 1 provides a set of XPS peaks corresponding to the various samples prepared, together with the best deconvolution into individual components. The characteristic hexagonal sp 2 arrangement expected for the Gr-based materials under study was determined by high-resolution transmission electron microscopy (TEM) and selected area electron diffraction. Figure 1 presents representative TEM images for two of these samples showing that they exhibit hexagonal ordering domains and intense hexagonal electron diffraction patterns, indicating a high degree of structural arrangement of the samples at the microscopy level. Figure 1: Microscopy images. TEM ( a , scale bar 500 nm) and HR-TEM ( b , scale bar 5 nm) images recorded for (P)Gr showing the sample layer morphology from the contrast with the background, the characteristic wrinkles, the ordering and arrangement at the atomic level. Full size image The monolayer or few-layer morphology of the Gr-based samples suspended in water, ethanol and halogenated solvents was assessed using atomic force microscopy (AFM) images with subnanometric vertical resolution. 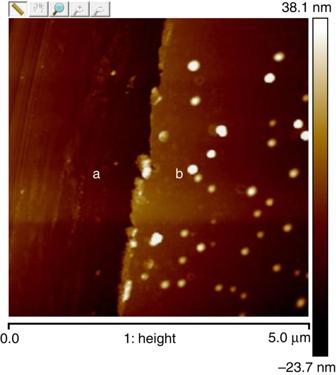Figure 2: AFM image. AFM of (N)Gr sheet (a) that is 1 nm in height with respect to the support (b). The white spots correspond to some nanoparticles and debris deposited on the single-layer graphene. Figure 2 shows selected AFM images of the Gr-based materials prepared and tested as hydrogenation catalysts in this work. It should be commented that some of the catalytic tests have been performed with powdered samples that have been obtained by freeze-drying water removal of Gr suspensions prepared by ultrasound exfoliation. In this case, the lyophilized solid samples should have a variable degree of stacking of the graphenic layers and cannot be strictly denoted as Gr, since the monolayer or few-layer morphology may have no sense in the solid state. The poor stacking of the Gr layers in the lyophilized powder was confirmed with X-ray diffraction that shows a very broad diffraction peak centred at 2Θ 27° characteristic of graphitic carbon residues with a disordered and loose stacking of the layers. Figure 2: AFM image. AFM of (N)Gr sheet ( a ) that is 1 nm in height with respect to the support ( b ). The white spots correspond to some nanoparticles and debris deposited on the single-layer graphene. Full size image Thermoprogrammed hydrogen desorption (TPD) The Gr-based materials under study were initially screened to determine their ability to interact with hydrogen gas. Two sets of experiments wherein Gr materials were exposed to hydrogen at room temperature or at 120 °C were performed, and after removal of the weakly physisorbed hydrogen by flushing argon at room temperature for 20 min the samples were heated at increasing temperatures. It was observed that the uptake of hydrogen increases significantly with the temperature of hydrogen adsorption, and values of hydrogen uptake of 0.22 and 1.02 mmol × g −1 were obtained for Gr upon adsorption of hydrogen at room temperature or 120 °C, respectively. Desorption profiles are presented in the Supplementary Fig. 2 and show that hydrogen is strongly bound to Gr and starts to desorb at ~650 °C, having a peak at 730 °C. These temperature values indicate that hydrogen should be forming covalent bonds with the graphenic sheets. Attempts to characterize these C–H bonds spectroscopically have met with failure so far. Raman spectroscopy did not detect changes in the sample probably because of the low sensitivity of this spectroscopy for C–H bonds. Fourier transform infrared spectroscopy is also not suitable because of the black colour of the samples and the difficulty to prepare self-supported wafers of sufficient transparency or reflectance. Overall, the hydrogen TPD measurements indicate that our samples do interact strongly with hydrogen, as it should be considering the abundant precedents in the formation of graphane from Gr materials that have been characterized mainly by the associated electrical conductivity decrease compared with Gr [33] . It is very likely, however, that the strongly bound hydrogen is not the one catalytically active in hydrogenation reactions and that only the fraction of the total chemisorbed hydrogen that is activated but loosely bound to Gr is the one that is mechanistically relevant. Catalytic gas-phase hydrogenation of acetylene and ethylene The Gr-based materials of Table 1 were tested as carbocatalysts for the selective hydrogenation of acetylene in the presence of a larger amount of ethylene at temperatures ranging from room temperature to 150 °C in a stream containing three times excess of hydrogen with respect to the amount of acetylene. Nitrogen was used as carrier gas. These mixtures of ethylene with small proportions of acetylene are of high relevance in petrochemistry, since they correspond to some of the ethylene streams, the target being the selective hydrogenation of acetylene to ethylene avoiding costly purification and minimizing the risks and complications associated with the presence of acetylene [34] , [35] . There are several patents describing the selective acetylene hydrogenation as a valid approach to tackle with this problem [36] , [37] , [38] . Importantly, all the Gr-based materials exhibit activity as hydrogenation catalysts even at room temperature, although obviously the optimal conditions were found at higher temperatures. Starting at room temperature using Gr as catalyst ( Supplementary Tables 1 and 2 ), preferential acetylene hydrogenation in the presence of the excess of ethylene was observed, reaching a conversion of 16%. This activity is remarkable considering the low reaction temperature and that hydrogenation is carried out under continuous flow. Hydrogenation of acetylene on frustrated Lewis acid–base pairs using a rigid amino–borane molecular catalyst has been reported in the literature [39] , and now the finding that Gr-based materials can also act as acetylene hydrogenation catalysts can open new opportunities in the area of metal-free hydrogenation catalysts. The conversion of acetylene in the presence of Gr as catalyst increases along the temperature, reaching an optimal value at temperatures between 110 and 120 °C, in which 99% of acetylene was converted with only 21% conversion of ethylene ( Table 2 , entry 2). Upon further temperature increase, selectivity of the acetylene versus ethylene hydrogenation decreases significantly. Besides Table 2 , Supplementary Tables 1–9 compile extensive data of selective acetylene hydrogenation in the presence of ninefold higher proportion of ethylene under other reaction conditions. It is worth remarking that GO is able to achieve at 150 °C 50.6% of acetylene conversion with no measurable ethylene hydrogenation ( Supplementary Table 4 ), while rGO reaches at 130 °C almost complete acetylene conversion with only 5.0 ethylene hydrogenation ( Supplementary Table 6 ). 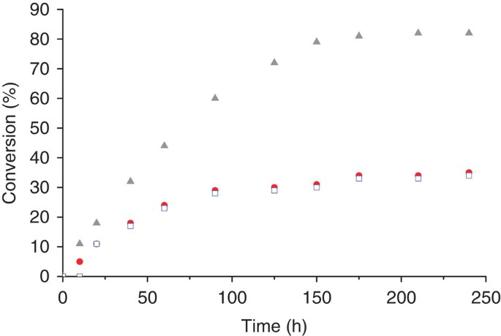Figure 4: Reaction kinetics. The time-conversion plot for hydrogenation of cyclooctene on Gr and rGO using different catalyst loadings. Full circle, 7 mg Gr; empty square, 7 mg rGO; full triangle, 40 mg Gr. Table 2 Catalytic results. 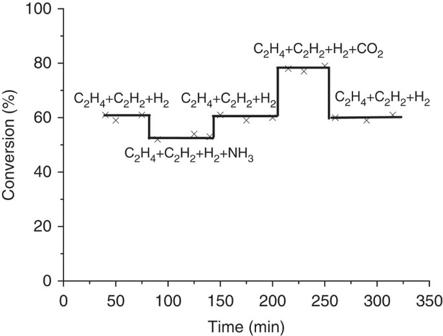Figure 6: Influence of acidic and basic gases. Time on stream of acetylene conversion at 100 °C in the presence of Gr as catalyst. Conditions: catalyst Gr: 7 mg, 100 °C, flow 1.7 ml × min−1of acetylene 1%, ethylene 9%, H23% and 15.2 ml × min−1of N2. First step: pure N2; second step: N2+10% NH3; third step: pure N2; fourth step: N2+10% CO2; fifth step: pure N2. Full size table To put these results into context, it should be mentioned that selective hydrogenation of similar mixtures of acetylene and ethylene have been recently reported using ceria as catalyst at temperatures above 200 °C, reaching lower conversions and acetylene selectivity under much higher hydrogen pressure [40] . To provide a valid comparison with the performance of Gr materials with respect to that of transition metals typically used as hydrogenation catalysts, the catalytic activity of Pt, Pd and Ni supported on active carbon at 1 wt % loading was also determined under the same reaction conditions. The results are provided in Supplementary Tables 10–12 . As it can be seen there, Pt/C and Pd/C are efficient catalysts for the hydrogenation of acetylene, Ni/C exhibiting lower activity. However, the percentage of fully hydrogenated ethane is remarkable in the case of Pt/C and Ni/C reaching over 20%, while the three metal catalysts afford a significant percentage of polymerization. Full hydrogenation to ethane and polymerization are undesirable processes that may accompany the selective acetylene hydrogenation. Overall, the results of the selective hydrogenation of acetylene in the presence of ethylene using Gr materials shows a catalytic activity that is comparable or even better than Pt/C, Pd/C and Ni/C. In addition to the excellent performance of Gr and rGO, the most salient features of Table 2 and Supplementary Tables 1–9 are the general hydrogenation activity of all Gr materials and the remarkable influence of the structure and doping of Gr on the performance of Gr material in this process. Concerning the product distribution of acetylene/ethylene hydrogenation, besides ethylene and very minor ethane proportion arising from acetylene and ethylene hydrogenation, a series of C 4 hydrocarbons and higher oligomers (C 4 +) were also observed, particularly upon increasing the temperature around 110 °C or above (see Supplementary Tables 4 and 6 ). Thus, rGO and GO were found very selective with respect to acetylene conversion; however, the product distribution indicates for both catalysts the formation of a large proportion of C 4 hydrocarbons. The similar catalytic performance, but lower activity of GO, is understandable considering that GO should undergo in situ hydrogen reduction under the reaction conditions rendering rGO. The series of heteroatom-doped Grs exhibit significantly lower activity than Gr or rGO, a fact that indicates that dopant elements are not the main active sites in hydrogenation. (N)Gr and (S)Gr perform similarly in the process, the important feature of the product distribution being in this case the appearance of C 4 + oligomers, the highest selectivity for C 4 + being observed for (S)Gr ( Supplementary Table 9 ). It is notable that in the case of (N)Gr formation of these C 4 + oligomers takes place even at room temperature ( Supplementary Table 7 ), and its selectivity remains relatively constant in the range of temperatures studied. The influence of doping on the selectivity of the reaction constitutes a notable example of how the activity and selectivity of a carbocatalyst can be controlled. 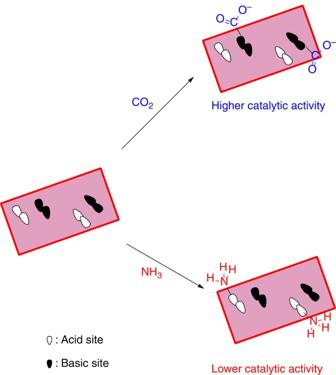Figure 7: Frustrated Lewis acid–base pairs. Proposal to rationalize the influence of CO2and NH3on the catalytic activity of Gr based on the interaction with basic and acid sites, respectively. Concerning dimerization/oligomerization accompanying hydrogenation, controls showed that no dimerization/oligomerization takes place in the absence of hydrogen. Since in the presence of hydrogen acetylene conversion is always high, it is reasonable to assume that dimerization/oligomerization is a process that accompanies acetylene hydrogenation, probably having common reaction intermediates. To understand this phenomenon better and to assess the stability of the Gr-based materials, we performed Raman and XP spectroscopies of the Gr materials after being used as catalysts. No changes were observed in the spectra of the most active Gr and rGO catalysts with respect to the fresh samples. As expected, it was observed that GO becomes converted into rGO. In the case of (N)Gr, it was clearly observed using XPS that nitrogen atoms are removed from the sample. Interestingly, the removal of nitrogen was observed upon the use of (N)Gr as hydrogenation catalyst or by direct treatment of the (N)Gr with hydrogen at 120 °C in the absence of acetylene and ethylene. It is noticeable that the removal of N is accompanied by the appearance of a new band with the binding energy of 285.8 eV that is typical for the C sp 3 species ( Supplementary Fig. 1 ) [32] . These results may indicate that the hydrogenation removes nitrogen from (N)Gr by formation of ammonia and partially hydrogenated Gr resulting in sp 3 carbon atoms. To support this hypothesis, we treated (N)Gr with a hydrogen flow in the absence of acetylene and ethylene under the same reaction conditions, whereby the removal of N by XPS was observed again ( Supplementary Fig. 1 ). Trapping with sulfuric acid reveals that NH 3 is formed in the process. Interestingly, the catalytic activity of denitrogenated (N)Gr H2 is similar to that of (N)Gr. This could be interpreted assuming that (N)Gr undergoes fast denitrogenation under the reaction conditions, and then the observed catalytic activity really corresponds to the denitrogenated (N)Gr H2 material. It could be that these defects generated by denitrogenation of (N)Gr are the sites responsible for the unique selectivity of (N)Gr towards C 4 + oligomers under hydrogenation conditions. The stability study also revealed that for (P)Gr ~65% and for (S)Gr all the dopant element remain unaltered after being used as the material in the selective hydrogenation of acetylene at 150 °C. Supporting information presents a comparison of the Raman and XP spectra of these materials before and after being used as catalysts ( Supplementary Figs 1 and 3 ). Besides spectroscopic techniques, stability of the two most active samples, Gr and rGO, was also assessed with TEM. It was observed that after prolonged use as catalysts at 150 °C, Gr and rGO powders were recovered from the reactor and suspended by sonication in methanol. TEM imaging of these two samples shows that the 2D morphology characteristic of Gr and the hexagonal arrangement have been preserved during the use of these solids as hydrogenation catalysts ( Supplementary Fig. 4 ). Role of metal impurities as hydrogenation-active sites Gr materials used as hydrogenation catalysts have two different precursors ( Table 1 ). Either they were obtained by pyrolysis of biopolymers presumably naturally exposed to very minor concentrations of transition metals or they were obtained by chemical oxidation of graphite with an excess of KMnO 4 . It could, then, be possible that the presence of metals in trace amounts could be responsible for the catalytic activity in acetylene–ethylene hydrogenation. To address the possible role of metal impurities, GO was selected since this sample is the one that contains metal impurities in higher concentration. It has been reported in the literature that rGO contains metallic impurities present in parent graphite and that they interfere in the electrochemistry of rGO [41] . Reported chemical analysis has revealed that GO obtained by Hummers oxidation may contain Fe (529.6 p.p.m. ), Ni (5.2 p.p.m. ), Cu (3.5 p.p.m.) and Mo (1.5 p.p.m.) among other elements [42] . We also performed qualitative analysis of the parent graphite and GO. We observed the presence of trace amounts of Fe and Ni (very minor) in graphite and Mn (major), Fe and Ni (minor) in GO. The presence of S was also detected in GO. Quantitative chemical analysis of GO indicates that the concentrations of Mn and Fe are 150±23 and 8±2 p.p.m.’s, respectively. To rule out the possible role of metal impurities in the catalytic activity of Gr, two alternative strategies were followed. In one of them GO was submitted to purification by dialysis to remove as much soluble metal ions as possible, the resulting GO sample having ~60% less Mn (58±9 p.p.m.) still exhibiting the expected catalytic activity ( Supplementary Table 13 ). In a second strategy, GO was impurified on purpose with two known amounts (5 and 10 p.p.m.’s) of MnCl 2 or PdCl 2 and then submitted to reduction to obtain impurified rGO. Unexpectedly, it was found that Mn impurification decreases the hydrogenation activity of rGO, notably the threshold temperature to observe acetylene hydrogenation ( Supplementary Tables 14 and 15 for 5- and 10-p.p.m. Mn impurification, respectively). In contrast, the presence of Pd increased a little acetylene conversion with respect to the plain rGO sample ( Supplementary Tables 16 and 17 ). A possible explanation is that, while Mn is devoid of activity as hydrogenation catalyst and its presence blocks some Gr-active sites, Pd has intrinsic activity as hydrogenation centres at these concentrations. However, extrapolation of the activity at 0 p.p.m. Pd concentration for temperatures of 90 °C or above reveals that GO should have catalytic activity per se, since the values are almost coincident to those measured for rGO. In summary, chemical analysis reveals that GO contains detectable amounts of transition metals; however, the catalytic data obtained after purification or impurification of GO at the p.p.m. 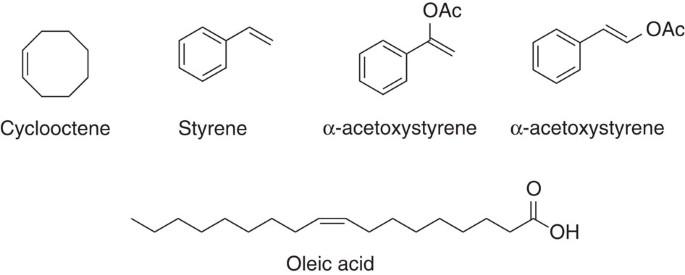level are in favour of the intrinsic catalytic activity of GO. Liquid-phase hydrogenation of C=C bonds To show the general applicability of Gr materials, particularly rGO and Gr, as carbocatalysts for hydrogenation reactions, we also studied the hydrogenation in the liquid phase under batch conditions at moderate temperatures and pressure of cyclooctene, three representative styrenes and oleic acid ( Fig. 3 ). Figure 3: Chemical structures. Structure of the alkenes submitted to hydrogenation in the presence of Gr catalysts. Figure 3: Chemical structures. Structure of the alkenes submitted to hydrogenation in the presence of Gr catalysts. Full size image Exfoliation by sonication in the corresponding solvent (heptanes or mesitylene) results in the formation of single- or few-layer Gr material as it has been proved previously and is documented in the literature [29] , [30] , [31] . In every case, except for β-acetoxystyrene, the reaction proceeds in a large extent, reaching complete conversion at sufficiently long reaction times ( Supplementary Tables 18 and 19 ). Controls with cyclooctene in which no Gr was added, Gr powder was added but the suspension was not sonicated failed to afford cyclooctane, indicating that neither the reactor nor carbonaceous Gr powders act as hydrogenation catalysts. In all cases, the only product observed was the expected compound of alkene hydrogenation. It was observed that the catalytic activity order of the Gr materials follows the same order already found for the selective acetylene hydrogenation, the most efficient catalysts being Gr and rGO. As an example, Fig. 4 shows the time-conversion plot for the hydrogenation of cyclooctene by Gr and rGO. Figure 4: Reaction kinetics. The time-conversion plot for hydrogenation of cyclooctene on Gr and rGO using different catalyst loadings. Full circle, 7 mg Gr; empty square, 7 mg rGO; full triangle, 40 mg Gr. Full size image Hydrogenation of styrene, α-acetoxy- and β-acetoxystyrene occurred selectively to the alkene group using Gr as the catalyst with a conversion of 76.7%, 82.1% and 9.1%, respectively. These results indicate that Gr is also able to catalyse hydrogenation of conjugated C=C double bonds. The difference in reactivity between α- and β-acetoxystyrene reflects the influence of steric hindrance on the C=C on the reactivity of the substrate, as it is also found in conventional noble metal catalysis in which substitution influences the relative reactivity of the substrates [43] , [44] . Reaction mechanism There are examples in the literature showing that discrete molecules comprising Lewis acid–base pairs separated at a distance that they do not undergo neutralization (‘frustrated Lewis acid–base pairs’) can activate hydrogen and act as hydrogenation catalysts [21] , [45] , [46] , [47] , [48] , [49] , [50] . On the basis of this known activity of frustrated Lewis acid–base pairs in organic molecules acting as metal-free hydrogenation catalysts, a reasonable proposal to rationalize the catalytic activity of Gr materials as hydrogenation catalysts would be the existence on the Gr layer of similar type of frustrated Lewis acid–base pairs consisting of the case of Gr by independent acid and basic pairs located on the Gr sheet at an adequate distance to promote the splitting of H 2 molecules. Then, activation of H 2 on Gr would take place as it occurs in the type of molecules having frustrated Lewis acid–base pairs by polarization of H 2 with the simultaneous formation of H + -like and H − -like sites. We have shown before experimental evidence based on H 2 -TPD of the strong interaction of Gr materials with hydrogen. Accordingly, it seems that the reaction mechanism should involve the uptake of H 2 on the Gr sheet that subsequently would transfer to the organic substrate having multiple C–C bonds. This claim was further supported by pre-adsorbing D 2 on Gr, followed by evacuation and heating with a H 2 stream, whereby the presence of H–D was detected with mass spectrometry ( Supplementary Fig. 6 ). To support the present claims, we proceeded to perform independent titrations of Gr and (N)Gr with NH 3 and CO 2 to quantify the presence of acid and basic sites, respectively. A summary of the desorption profiles with the temperature is shown in Supplementary Fig. 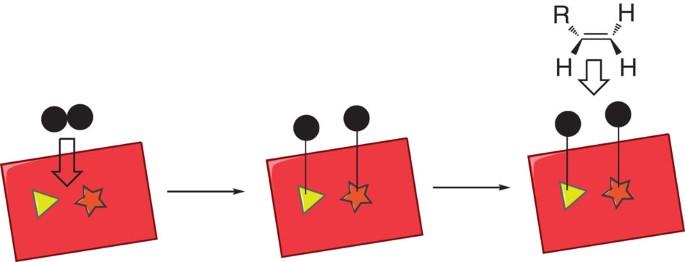5 . The results obtained, in fact, allow to determine and quantify the presence on these Gr materials of both acid and basic sites, some of which are relatively strong since, for instance, CO 2 desorption on Gr exhibits a peak at 680 °C, corresponding to basic sites of high strength. Figure 5: Reaction mechanism. Proposal to rationalize the activity of Gr materials as hydrogenation catalysts based on the presence of frustrated Lewis acid–base sites. Triangle and star represent the acid and basic sites, respectively, on the Gr sheet at a certain distance suitable by react with H2molecules (as black spheres). These active hydrogen atoms on the Gr surface will be subsequently transferred to the alkene. Figure 5 summarizes our proposal. Figure 5: Reaction mechanism. Proposal to rationalize the activity of Gr materials as hydrogenation catalysts based on the presence of frustrated Lewis acid–base sites. Triangle and star represent the acid and basic sites, respectively, on the Gr sheet at a certain distance suitable by react with H 2 molecules (as black spheres). These active hydrogen atoms on the Gr surface will be subsequently transferred to the alkene. Full size image To further confirm the involvement of both acid and basic sites on Gr in the catalytic hydrogenation, control experiments in which the selective acetylene hydrogenation was carried out in a stream containing CO 2 or NH 3 were carried out. The reaction conditions selected (100 °C) allowed the observation of negative or positive effects of these gases, by increasing or decreasing acetylene conversion. It was found that acetylene conversion depends on the presence of CO 2 (increasing conversion by 33%) or NH 3 (decreasing conversion by 9%) in the stream. These effects were reversible and the catalytic activity of Gr was recovered to the initial state in the absence of CO 2 or NH 3 , when these gases were removed. This indicates that, under the reaction conditions, the interaction of CO 2 and NH 3 with the active sites was of Gr not irreversible. Figure 6 presents the time on the stream plot of acetylene conversion in these experiments in the presence of CO 2 and NH 3 , while Supplementary Fig. 7 presents the change noticed in the selectivity of ethane formation in the presence of these gases. Figure 6: Influence of acidic and basic gases. Time on stream of acetylene conversion at 100 °C in the presence of Gr as catalyst. Conditions: catalyst Gr: 7 mg, 100 °C, flow 1.7 ml × min −1 of acetylene 1%, ethylene 9%, H 2 3% and 15.2 ml × min −1 of N 2 . First step: pure N 2 ; second step: N 2 +10% NH 3 ; third step: pure N 2 ; fourth step: N 2 +10% CO 2 ; fifth step: pure N 2 . Full size image Although a conceptual framework is needed to understand the process and complete quenching of the reaction was not observed, the activity data shown in Fig. 6 strongly support the influence of acid and basic sites on the conversion. A plausible explanation of the activity data could be that carboxylate-like groups generated by reaction of CO 2 with basic sites promote the reaction in combination with the acid sites neutralized by NH 3 . Figure 7 summarizes the proposal. Other possibilities, such as interaction of NH 3 with the quinone-like groups, although less likely to be reversible under the operation conditions, can, however, not be ruled out with the present data. Further mechanistic studies combined with in situ characterization techniques and modelling are necessary to determine the structure of the sites that activate molecular H 2 as well as to provide information about the homolytic versus the heterolytic cleavage of the H–H bond. Figure 7: Frustrated Lewis acid–base pairs. Proposal to rationalize the influence of CO 2 and NH 3 on the catalytic activity of Gr based on the interaction with basic and acid sites, respectively. Full size image With respect to the role of the dopant element on the activity, the catalytic data indicate that they exert influence on the product distribution, rather than in the acetylene conversion. Thus, their role in hydrogen activation seems to be secondary for the samples under study. It appears that the presence of heteroatoms or the defects created after their complete or partial removal are more likely to interact with the organic intermediates, favouring their addition on ethylene forming dimers. Theoretical calculations and surface techniques are necessary to gain full understanding on this issue. The above data show that Grs in the absence of any transition metal are general catalysts for the hydrogenation of multiple C–C bonds, both in the gas phase and in the liquid phase. The results obtained also show that these Gr materials can be selective catalysts for acetylene hydrogenation in the presence of large excess of ethylene by optimizing the temperature and composition of the catalyst. The presence of dopant elements notably influences the activity and selectivity of the materials, promoting the formation of dimers and oligomers. Gr can also act as hydrogenation catalysts in the liquid phase for isolated and conjugated C=C bonds, the reaction being sensitive to the steric encumbrance around the group. Considering that hydrogenation reactions is a paradigmatic reaction catalysed by noble, precious metals, the present report can contribute to the application of metal-free catalysts for this reaction. Preparation of GO Graphite flakes (3 g) were suspended in a mixture of concentrated H 2 SO 4 /H 3 PO 4 (360:40 ml). To this mixture, KMnO 4 (18 g) was added by producing an exothermic reaction raising the temperature to 35–40 °C. This reaction mixture was then heated to 50 °C under stirring for 12 h. The reaction was cooled to room temperature and poured into 400 g of ice containing 30% H 2 O 2 (3 ml). After air-cooling, the suspension was filtered, washed with 1:10 HCl (37%) solution and then further washed with water. The remaining solid was sonicated with 400 ml of water for 30 min and centrifuged at 4,000 r.p.m. for 4 h. The supernatant was centrifuged at 15,000 r.p.m. for 1 h. The solid obtained, after centrifugation at 15,000 r.p.m., was dried at 60 °C. Qualitative chemical analysis of metals at trace impurity levels was performed with X-ray fluorescence of parent graphite and GO powders without any pretreatment. Quantitative chemical analysis of the metal impurities was performed, suspending a known weight of GO powder in concentrated aqueous HCl solution for 1 day and analysing by inducitvely coupled plasma (ICP) the Mn, Fe, Ni and Cu content. One sample of GO was submitted to dialysis using commercial cellulose membrane (Aldrich D6191, molecular weight cutoff 12,000). The aqueous suspension of GO (100 ml, 5 mg ml −1 ) was introduced inside the membrane that was immersed inside a vessel containing 1 l of milliQ water. The system was magnetically stirred at room temperature for 4 days, the milliQ water being replaced each day. After dialysis, the membrane was taken and the resulting GO recovered with lyophilization. The four aliquots of milliQ water were combined and submitted to ICP chemical analysis. Preparation of rGO rGO was prepared by hydrothermal reduction of GO in the absence of any chemical. Briefly, 100 ml of an aqueous suspension of GO (5 mg ml −1 ) was introduced in a Teflon-lined autoclave and heated at 180 °C for 3 h. After this time, the suspension was centrifuged at 15,000 r.p.m. for 1 h and the resulting rGO solid at the bottom of the tube was collected. Impurification of rGO by MnCl 2 and PdCl 2 was carried out by adding purposely 5.7 or 11.5 μg of MnCl 2 or 8.4 or 11.5 μg of PdCl 2 during the preparation of rGO. This leads to 5 or 10 p.p.m.’s Mn or Pd impurified rGO. The required amount of MnCl 2 or PdCl 2 was dosed by adding with a syringe 100 μl of a solution containing 5.7 or 11.5 mg ml −1 of MnCl 2 or 8.4 or 11.5 mg ml −1 of PdCl 2 , respectively. Chemical analysis of the aqueous solution after removal of rGO did not detect the presence of Mn or Pd in the supernatant, indicating a complete adsorption of the inorganic salts on rGO. Synthesis of Gr Alginic acid sodium salt from brown algae (Sigma) was pyrolized in the argon atmosphere using the following oven programme: 200 °C during 2 h for annealing and then heating at 10 °C min −1 up to 900 °C for 6 h. This multilayer Gr powder is sonicated at 700 W during 1 h to obtain the dispersed Gr in the reaction mixture. Synthesis of N-doped Gr Chitosan from Aldrich (low molecular weight) was pyrolized in the argon atmosphere using the following oven programme: 200 °C during 2 h for annealing and then heating at 10 °C min −1 up to 900 °C for 6 h. This multilayer Gr powder is sonicated at 700 W during 1 h for obtaining the dispersed (N)Gr in the reaction mixture. Synthesis of P-doped Gr Alginic acid sodium salt (0.5 g) from brown algae (Sigma) was dissolved in a sodium phosphate dibasic monohydrate aqueous solution (0.2 g in 50 ml of water). The solutions were filtered in a pressure filtration equipment using 0.22-μm-pore diameter filters for removing the impurities present in commercial alginate. Before pyrolysis, the solution was concentrated by heating in an oven at 100 °C overnight. Pyrolysis was performed using the same oven programme as indicated for the preparation of Gr. During the process, formation in the walls of elemental red P was observed. The resulting graphitic powder was sonicated at 700 W during 1 h in water to obtain (P)Gr dispersed in the reaction mixture. Synthesis of S-doped Gr λ-Carragenan (Sigma) was pyrolized in the argon atmosphere using the following oven programme: 200 °C during 2 h for annealing and then heating at 10 °C min −1 up to 1,000 °C for 6 h. This multilayer Gr powder is sonicated at 700 W during 1 h to obtain the dispersed (S)Gr in the reaction mixture. Metal-loaded carbon Pt/C and Pd/C at 1 wt% metal loading were commercial catalysts (Aldrich). Ni/C was prepared by suspending 1 g of Norit active carbon in 100 ml water and addition of 205 mg of Ni(NO 3 ) 2 under magnetic stirring at room temperature. The suspension is stirred for 1 h, filtered and then dried in an oven at 60 °C. The resulting Ni-containing active carbon was reduced for 2 h at 200 under H 2 stream before using the material as catalyst. Catalytic tests The performance of the Gr-based catalysts was studied in the hydrogenation of an acetylene (10%)–ethylene (90%) gas mixture, of cyclooctene, three styrenes and oleic acid. Hydrogenation of the acetylene (10%)–ethylene (90%) gas mixture (provided by Linde Gas) was carried out using a fixed-bed tubular stainless-steel microreactor (length of 300 mm and i.d. of 9 mm) system from PID&ENG equipped with a thermocouple in the middle of the catalyst bed. The catalyst (7 mg) was placed between two layers of quartz wool. A gas mixture composed of acetylene (10%)–ethylene (90%), hydrogen (99.999%, provided by Linde Gas) and nitrogen (99.999%, provided by Linde Gas) with a molar ratio C 2 H 2 :H 2 :N 2 of 1:3:90 was fed with a total flow of 17.4 ml min −1 . The hydrogenation reactions were performed in range of temperature from ambient till 150 °C. Reactant and product streams were analysed using an online gas chromatograph (GC, Shimadzu 2014) equipped with a RT-Silica Bond capillary (50 m, 0.2 mm) connected to flame ionization detector for the analyses of hydrocarbons and Poropak-Q and RT-Msieve 5A columns (provided by the Restek) connected to a thermal conductivity detector for the analysis of permanent gases. Conversions were calculated based on the calibration curves established from the dependency of the chromatographic areas as a function of concentration and using the following equations: The batch experiments were carried out in a 16-ml autoclave with a stirrer from HEL. Typical catalytic conditions for considered 26 mg cyclooctene, 5 ml heptane, 80 °C, 4 h, 7 mg catalyst, 1,400 r.p.m., 30 bar H 2 for the case of hydrogenation of cyclooctene. In the case of the three styrene hydrogenations, the reaction was performed by dissolving 25 mg in 5 ml heptanes and the reaction carried out at 80 °C for 4 h using 7 mg of catalyst and stirring the reaction at 1,400 r.p.m. under 30 bar H 2 . For hydrogenation of oleic acid, 282 mg oleic acid were dissolved in 5 ml mesitylene, and the reaction carried out at 300 °C for 9 h using 30 mg catalyst stirring the reaction mixture at 1,400 r.p.m. under 30 bar H 2 . The liquid products were analysed using a gas chromatograph (Shimadzu GC-2014) equipped with a flame ionization detector and a capillary column DB-5 (length, 60 m; internal diameter, 0.32 mm; film thickness, 0.5 mm). In the case of oleic acid, the following temperature programme was used for analysis: 313 K hold for 2 min and 523 K (5 K min −1 ) hold for 10 min. Samples were silylated with N,O-bis(trimethyl)-trifloroacetamide (BSTFA). BSTFA (15 μl) and pyridine (15 μl) were added to the sample (100 μl). After addition of the silylation agent, the samples were kept in an oven at 333 K for 30 min. The products were confirmed using gas chromatography–mass spectrometry, using a Trace GC 2000 system with MS detector (Thermo Electron Scientific 65 Corporation, USA) incorporating a TR-WAX capillary column. Nitrogen quantification The quantity of nitrogen in the (N)Gr sample was quantified from the amount of ammonia ions generated during treatment of the (N)Gr sample with hydrogen at 120 °C for 6 h. The gaseous feed was trapped into a sulfuric acid solution (1 N), which was then titrated by a standardized sodium carbonate (0.1 N) till a pH of 4.0. TPD measurements H 2 -TPD measurements were carried out using the AutoChem II 2920 station. The sample (7 mg), placed in a U-shaped quartz reactor with an inner diameter of 0.5 cm, was pretreated under Ar (Purity 5.0, from Linde) at 120 °C for 1 h and then exposed to a flow of 10% H 2 in Ar (from Linde) for 120 min at room temperature or at 120 °C. After that, the sample was purged with a flow of Ar (50 ml min −1 ) for 20 min at 25 °C in order to remove the weakly adsorbed species. TPD was then started, with a heating rate of 5 °C min −1 till 800 °C. The desorbed products were analysed with a TC detector. The H 2 desorbed, expressed as mmoles of H 2 per grams of catalyst, was determined using a calibration curve. CO 2 - and NH 3 -TPD measurements were carried out using the same AutoChem II 2920 station. The samples (3–5 mg), placed in a U-shaped quartz reactor with an inner diameter of 0.5 cm, were pretreated under He (Purity 5.0, from Linde) at 120 °C for 1 h and then exposed to a flow of NH 3 or CO 2 (from SIAD) for 1 h. After that, the sample was purged with a flow of He (50 ml min −1 ) for 20 min at 25 °C in order to remove the weakly adsorbed species. TPD was then started, with a heating rate of 10 °C min −1 till 850 °C. The desorbed products were analysed with a TC detector. The desorbed NH 3 or CO 2 , expressed as mmols per grams of catalyst, was determined using a calibration curve. RAMAN spectroscopy Raman spectra were acquired using a Labram-HR (Horiba Jobin Yvon) Raman spectrometer (600 mm −1 grating, 100 μm entrance slit) coupled to a Peltier-cooled CCD detector (Andor DU420) and an Olympus BXFM optical microscope. Raman scattering was excited at 632.8 nm by means of a HeNe laser with 0.1-mW excitation power on the sample. The laser beam was focused on the sample via a long-working distance × 50 microscope objective (numerical aperture=0.5), which served also to collect the scattered photons. The Rayleigh scattering was removed by a holographic notch filter and the Raman spectra were recorded between 200 and 2,000 cm −1 . XPS measurements The XPS measurements were recorded with a spectrometer (manufactured by Specs, Germany), which operates with a monochromatized AlK α1 radiation (1,486.74 eV) and a 150-mm Phoibos hemispherical electron energy analyser. For the calculation of the binding energies, the C 1 s peak of the C–(C,H) component at 284.8 eV was used as an internal standard. The data are analysed by fits with Voigt profiles and computing their integrals. The binding energies assigned to the C 1 s , N 1 s , P 2 p , S2 p , O1 s levels were analysed. Isotopic H/D scrambling measurements promoted by G A sample of 40 mg of Gr was evacuated at 10 −3 mbar and then D 2 was introduced at a pressure of 0.5 bar. The system was maintained at room temperature for 24 h. Then the sample was introduced one line in a chromatographic column connected to a SMQuadrupolar analyzer and the temperature was increased at 100 °C, while the sample was flused with flow of argon (10 ml min −1 ) monitoring the m/z masses of 2 (H 2 ), 3(HD), 4 (D 2 ) and 40 (Ar) till stabilization. After stabilization and a second evacuation, a flow of 8 ml min −1 Ar and 2 ml min −1 H 2 was passed over the sample checking following the same m/z components 2(H 2 ), 3(D 2 ) and 4(D 2 ). The results are presented in Supplementary Fig. 6 . How to cite this article: Primo, A. et al. Graphenes in the absence of metals as carbocatalysts for selective acetylene hydrogenation and alkene hydrogenation. Nat. Commun. 5:5291 doi: 10.1038/ncomms6291 (2014).